TMC-1 attenuatesC. elegansdevelopment and sexual behaviour in a chemically defined food environment Although diet affects growth and behaviour, the adaptive mechanisms that coordinate these processes in non-optimal food sources are unclear. Here we show that the C. elegans tmc-1 channel, which is homologous to the mammalian tmc deafness genes, attenuates development and inhibits sexual behaviour in non-optimal food, the synthetic CeMM medium. In CeMM medium, signalling from the pharyngeal MC neurons and body wall muscles slows larval development. However, in the non-standard diet, mutation in tmc-1 accelerates development, by impairing the excitability of these cells. The tmc-1 larva can immediately generate ATP when fed CeMM, and their fast development requires insulin signalling. Our findings suggest that the tmc-1 channel indirectly affects metabolism in wild-type animals. In addition to regulating the development, we show that mutating tmc-1 can relax diet-induced inhibition of male sexual behaviour, thus indicating that a single regulator can be genetically modified to promote growth rate and reproductive success in new environments. An animal’s behaviour and ability to metabolize novel nutrients are traits that can be modified by evolution [1] . Since diets affect the development and reproduction [2] , [3] , organisms must sense their nutritional environment and their metabolic state and alter their physiological, behavioural and reproductive responses. Genetic changes that modify these processes allow organisms to invade and thrive in new ecological niches; however, the molecules that can be altered to achieve this aim remain unclear. C. elegans has been used to study how diet impacts gene expression, developmental rate, reproduction and lifespan [3] . C. elegans is a free-living bacterivore containing ~1,000 somatic cells, 60 of which form the pharynx and its associated neurons. The pharyngeal system pumps in, grinds up and transfers bacterial food into the intestine [4] . The laboratory diet for C. elegans is E. coli OP50. At 20 °C, worms develop from L1 larvae to adults in 3 days [5] . C. elegans can be fed other bacterial species [4] , [6] , and different food sources can affect feeding, development, reproduction and lifespan [6] , [7] , [8] . For example, when fed with the bacteria Comamonas sp. , C. elegans develop faster, lay fewer eggs and live shorter than when fed with OP50 (ref. 3 ). In contrast to the fast growth on a Comamonas sp. diet, C. elegans can also develop in bacteria-free axenic media, but at a reduced efficiency. C. elegans maintenance medium (CeMM) was developed as an axenic chemically defined food source [9] , [10] , which exclude variables associated with bacterial metabolism [10] , [11] . Although CeMM has glucose, vitamins, salts, amino acids, nucleic acids and other factors, animals develop slower and males mate poorly [10] , [12] . Thus, this food is either missing components or is hard to utilize, making it a suboptimal food source for wild-type C. elegans . Therefore, we asked whether an organism can be manipulated to better utilize this defined nutrient source. In this report, we utilize CeMM and C. elegans to investigate the relationships between diet, life history traits and the mechanisms involved in coordinating these processes with the potential to adapt in non-optimal food sources. We show that multiple character traits, required for adapting to changing environmental circumstances, can be promoted through one gene mutation. tmc-1 functions to retard growth on CeMM To address what genetic factors can be modified for adaption to new diets, we used CeMM as our nutritional paradigm. When fed OP50 at 20 °C, C. elegans develop from L1 larvae to adults in 3 days [5] . When grown on CeMM-infused agarose plates, animals developed slowly; ~10% of the larvae developed into adults after 8 days post hatching (d.p.h. ), and the remainder developed asynchronously afterwards ( Fig. 1a ). 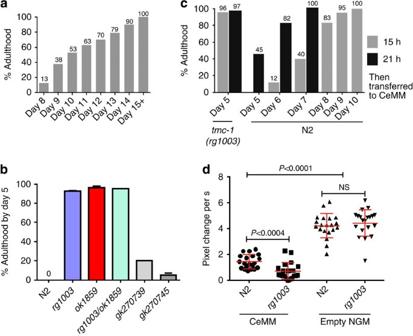Figure 1: Mutanttmc-1promotes fastC. eleganslarval development on CeMM. (a) Growth rate of wild-type N2 (n=100 worms; one trial), this represented the wild type growth rate on CeMM. (b)tmc-1mutants with different alleles developed faster than wild type on CeMM plates (n=30–100 worms; one for thetmc-1heterozygote; two trials for all others). (c) Growth rate on CeMM plates with 15 or 21 h OP50 culture from newly hatched L1 larvae (n=60 and 67, respectively; one trial). (d) Velocity of wild type andtmc-1(rg1003)on CeMM and empty plates (mean±s.d. of 20 animals; symbol represents single animal; Mann–Whitney non-parametric test). Figure 1: Mutant tmc-1 promotes fast C. elegans larval development on CeMM. ( a ) Growth rate of wild-type N2 ( n =100 worms; one trial), this represented the wild type growth rate on CeMM. ( b ) tmc-1 mutants with different alleles developed faster than wild type on CeMM plates ( n =30–100 worms; one for the tmc-1 heterozygote; two trials for all others). ( c ) Growth rate on CeMM plates with 15 or 21 h OP50 culture from newly hatched L1 larvae ( n =60 and 67, respectively; one trial). ( d ) Velocity of wild type and tmc-1(rg1003) on CeMM and empty plates (mean±s.d. of 20 animals; symbol represents single animal; Mann–Whitney non-parametric test). Full size image We screened for EMS (ethyl methanesulfonate)-generated mutants that developed the fastest on CeMM, and identified the rg1003 allele, which allowed 90% of larvae to develop into adults by 5 d.p.h. ( Fig. 1b ). Using two-point mapping and Illumina whole-genome sequencing, we mapped the rg1003 mutation to tmc-1 . The tmc-1 gene encodes a transmembrane channel-like (TMC) family protein [13] , [14] . tmc-1(rg1003) mutants develop normally when fed OP50 (that is, 3 days development from L1 larva to adult) and are grossly normal in morphology and behaviour, but some old hermaphrodites have defective egg-laying behaviour and reduced brood size ( Supplementary Fig. 1 ). tmc-1 is reported to promote sodium sensation and encodes a putative sodium-sensitive channel [15] , and the mammalian homologue is linked to deafness [16] , [17] , [18] . All TMC family proteins encode integral membrane proteins with at least six membrane-spanning domains [13] , [14] . tmc-1(rg1003) encodes a L367I change; this leucine is predicted to be in a transmembrane domain ( Supplementary Fig. 2 ) and is conserved in the mammalian TMC-1–4 and 7 proteins [14] . The rg1003 allele failed to complement the tmc-1(ok1859) deletion allele, which also induced rapid growth in CeMM ( Fig. 1b ). Mutants containing other tmc-1 alleles also developed faster in CeMM ( Fig. 1b ). When we examined the CeMM-fed animals’ developmental stages, we observed that tmc-1(rg1003) mutants developed into L3 larvae on day 3 and into L4 larvae on day 4 post hatching, whereas the wild type remained as L1 larvae during this period ( Supplementary Fig. 3 ). C. elegans also encodes an additional TMC protein, TMC-2; however, the CeMM-fed tmc-2(ok1302) deletion mutant does not display fast development (no adults by day 14, n =40). We asked if TMC-1 generally slows the development or retard a specific developmental stage. We found that regardless if the wild type or tmc-1(rg1003) L1 larvae were fed with bacteria up to ~L2 stage (15 h) or up to ~L3 stage (21 h), before being transferred to CeMM, the wild type always progressed through the larval developmental stages slower than the tmc-1 mutants ( Fig. 1c ). This indicated that TMC-1’s attenuation of growth is not limited to a developmental stage. We then asked if temporary growth on CeMM permanently alters the developmental rate. We grew the wild-type and tmc-1 mutants on CeMM for 48 h and then shifted them to OP50. We found that although the animals were at different developmental stages after CeMM feeding (the wild type was at early L1 stage, whereas tmc-1 mutants were late L1 to early L2, Supplementary Fig. 3 ), once they were introduced to OP50, both resumed the standard developmental rates [19] ( Supplementary Fig. 4 ). Since the tmc-1 mutants had a head start in development, the approximately late L1–L2 mutants took 23 h to reach the mid-late L4 stage, whereas the early L1 wild type had to develop through the L1 stage and they took 31 h of OP50 feeding to develop into mid-late L4. Thus, the data suggests that TMC-1’s function on growth is context dependent. TMC-1 was identified as a sodium-sensitive receptor/channel that is used on sensory neurons to detect environmental sodium [15] . Thus, we tested if increased sodium in the media accelerated or retarded development on CeMM or on NGM media, but found no changes on the wild-type or the tmc-1(rg1003) mutant’s development ( Supplementary Fig. 5a–c ). These data imply that TMC-1 might have other functions to regulate the cell physiology, in addition to the reported external sodium sensation. We next asked if tmc-1 mutants behave differently in CeMM. Previous studies found that locomotor activity is linked to an animal’s nutritional state; food-stressed animals seek food and increase exploratory behaviour, whereas food-satiated animals decrease exploratory behaviour [7] , [20] , [21] . We found that wild-type L1 larvae moved faster than tmc-1(rg1003) mutants on CeMM plates after 30 min of exposure, whereas on food-deprived NGM plates the locomotion rates for both groups of worms were much higher, but equivalent ( Fig. 1d ). The reduced tmc-1 mutant’s locomotion suggests that they acclimate to the CeMM plates better than the wild type. Next we checked other life history traits such as brood size, reproductive aging and life span on CeMM, and these traits were not affected by tmc-1(rg1003) ( Supplementary Fig. 6 ). TMC-1 slows growth through neurons and muscles tmc-1 was reported to be expressed in sensory neurons, cholinergic ventral cord neurons and additional unidentified head, motor and interneurons [15] , [22] . However, which of these TMC-1-expressing tissues regulate development was not obvious. To further identify tmc-1 -expressing cells, we expressed an 8.4-kb construct containing 3.6 kb upstream of the tmc-1 start site and the first exon to part of the third exon fused to YFP. In addition to the reported expression patterns, tmc-1 was expressed in body wall muscles ( Fig. 2a ), which is promoted by intronic DNA. The 3.6-kb promoter drives the expression in the reported ventral cord and head sensory neurons as-well-as SIBD, SIBV, ALA, AVH head neurons and I1, MC-pharyngeal neurons ( Fig. 2b,d and Supplementary Fig. 7 ), and the PHC neurons in the tail ( Fig. 2c ). 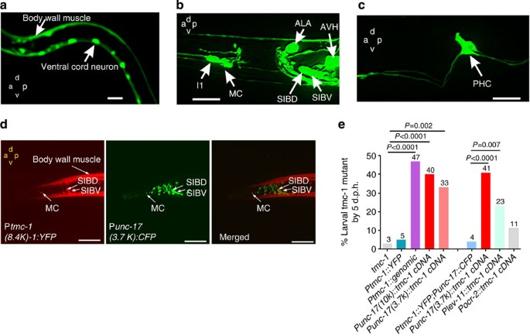Figure 2: TMC-1 attenuates development through cholinergic neurons and body wall muscles. (a–c) Additional identifiedtmc-1expression tissues through confocal Z-stack three-dimensional reconstruction. (a) The expression in body wall muscles in L1 larva. (b) The expression in I1, MC, SIBD, SIBV, ALA and AVH L1 head neurons, but not body wall muscles, because of intronic DNA in the expression construct. (c) The expression in PHC neurons in the tail of L4 larva. (d) Fluorescence image of the same animal showing co-labelling oftmc-1(8.4K)::YFP withunc-17(3.7k)::CFPin cholinergic SIBD, SIBV and MC neurons in L1 larva. (e) Transgenic rescue oftmc-1(ok1859)mutants on CeMM (n=37–77 worms; one trial; the four transgenes in the right are expressed in thepha-1;tmc-1(ok1859)background;Pvalues determined with Fisher’s exact test). A, anterior; D, dorsal; P, posterior; V, ventral. White arrows indicate expression in specified neurons or tissues. Scale bars, 10 μm. Figure 2: TMC-1 attenuates development through cholinergic neurons and body wall muscles. ( a – c ) Additional identified tmc-1 expression tissues through confocal Z-stack three-dimensional reconstruction. ( a ) The expression in body wall muscles in L1 larva. ( b ) The expression in I1, MC, SIBD, SIBV, ALA and AVH L1 head neurons, but not body wall muscles, because of intronic DNA in the expression construct. ( c ) The expression in PHC neurons in the tail of L4 larva. ( d ) Fluorescence image of the same animal showing co-labelling of tmc-1(8.4K) ::YFP with unc-17(3.7k)::CFP in cholinergic SIBD, SIBV and MC neurons in L1 larva. ( e ) Transgenic rescue of tmc-1(ok1859) mutants on CeMM ( n =37–77 worms; one trial; the four transgenes in the right are expressed in the pha-1;tmc-1(ok1859) background; P values determined with Fisher’s exact test). A, anterior; D, dorsal; P, posterior; V, ventral. White arrows indicate expression in specified neurons or tissues. Scale bars, 10 μm. Full size image The prominent regions that express tmc-1 are body wall muscles and cholinergic neurons; thus we tested if these cells moderated development on CeMM. We found that the wild-type tmc-1 promoter and genomic DNA suppress the tmc-1(ok1859) phenotype ( Fig. 2e ). To localize further the tmc-1 cell-specific function, we introduced tmc-1 cDNA with P unc-17(3.7k) , P unc-17(10k) and P lev-11(3.5k) promoters into the tmc-1(ok1859) mutant. unc-17 encodes a vesicular acetylcholine (ACh) transporter, and is expressed in cholinergic head/tail and ventral cord neurons [23] . lev-11 encodes muscle-expressed tropomyosin [24] . Strains expressing either the unc-17 or the lev-11 promoter constructs suppressed the tmc-1 phenotype, although the muscle-expressing transgene was less effective ( Fig. 2e ). We found that expression from either P unc-17(3.7k) or P unc-17(10k) promoters partially suppress the tmc-1(ok1859) phenotype ( Fig. 2e ). Thus, the data suggest that TMC-1 attenuates development through head cholinergic neurons and body wall muscles. TMC-1 slows growth via MC neurons The expression overlap between the P unc-17(3.7k) and the tmc-1 promoters suggest that the SIBD, SIBV and the MC-pharyngeal neurons ( Fig. 2d ) were candidates for further analysis. To address how the neurons regulate the tmc-1 -mediated response to CeMM, we expressed the Ca 2+ sensor GCaMP6 (ref. 25 ) from the neuron-specific P tmc-1(3.6k) promoter, to quantify differences in cytoplasmic Ca 2+ in the MC, SIBD, SIBV, ALA and AVH neurons, as a proxy for neural activity [26] . After 2 h of CeMM exposure, we found that in wild-type L1 larvae, the SIBD/V and ALA head neurons displayed a significant increase in steady-state Ca 2+ levels, relative to tmc-1(ok1859) larvae ( Fig. 3a ). Wild-type AVH and pharyngeal MC neurons steady-state Ca 2+ levels were also higher, but not statistically different ( Fig. 3a ). This suggests that in the wild type, the ALA and cholinergic SIBD/V neurons respond to the changes in the nutrient environment. The AVH head neurons and the pharyngeal MC neurons might also respond to CeMM, but the changes in their activities were too subtle to detect. 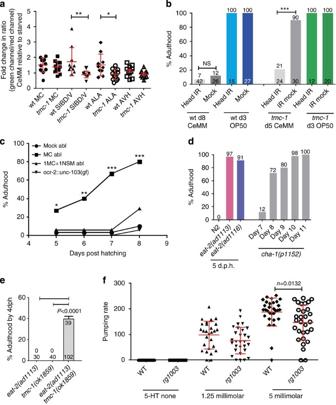Figure 3: TMC-1 retards growth via cholinergic transmission from MC to the pharyngeal muscles. (a)tmc-1(ok1859)L1 larvae mutants showed less calcium transient changes in SIBD/V and ALA after 2 h CeMM exposure, compared with starved than wild type (n=10–13 worms; symbol represents single animal; *P<0.05, **P<0.01, Student’st-test). (b) Growth rate of wild type andtmc-1(ok1859)L1 larvae with the posterior bulb areatmc-1-expressing neurons photoablated and then grown on CeMM or OP50 plates (nare listed on the bottom of the columns; NS: no significant statistical difference, ***P<0.001, Fisher’s exact test). (c) Laser ablation of the MC neurons in the wild type accelerated growth on CeMM (n=15–17 worms; *P<0.05, **P<0.01, ***P<0.001, Fisher’s exact test). (d) Growth rate of cholinergic mutants (n=30–100 worms). (e)eat-2;tmc-1double mutants grew faster than single mutants (nare listed on the bottom of the columns; Fisher’s exact test). (f) TMC-1 promoted MC neuronal excitability, the pumping response of wild-type N2 andtmc-1(rg1003)response to serotonin (n≥14; mean±s.d., symbol represents single animal; Mann–Whitney non-parametric test). Figure 3: TMC-1 retards growth via cholinergic transmission from MC to the pharyngeal muscles. ( a ) tmc-1(ok1859) L1 larvae mutants showed less calcium transient changes in SIBD/V and ALA after 2 h CeMM exposure, compared with starved than wild type ( n =10–13 worms; symbol represents single animal; * P <0.05, ** P <0.01, Student’s t -test). ( b ) Growth rate of wild type and tmc-1(ok1859) L1 larvae with the posterior bulb area tmc-1 -expressing neurons photoablated and then grown on CeMM or OP50 plates ( n are listed on the bottom of the columns; NS: no significant statistical difference, *** P <0.001, Fisher’s exact test). ( c ) Laser ablation of the MC neurons in the wild type accelerated growth on CeMM ( n =15–17 worms; * P <0.05, ** P <0.01, *** P <0.001, Fisher’s exact test). ( d ) Growth rate of cholinergic mutants ( n =30–100 worms). ( e ) eat-2;tmc-1 double mutants grew faster than single mutants ( n are listed on the bottom of the columns; Fisher’s exact test). ( f ) TMC-1 promoted MC neuronal excitability, the pumping response of wild-type N2 and tmc-1(rg1003) response to serotonin ( n ≥14; mean±s.d., symbol represents single animal; Mann–Whitney non-parametric test). Full size image When fed OP50, the MC neurons regulate pharyngeal pumping rate through secreting ACh to the pharyngeal muscles [4] , [27] ; SIB function is less clear, but is involved in the anterior nervous system organization [28] . Without tmc-1 , larvae develop faster in CeMM, so we hypothesized that removing tmc-1 -expressing cells might also accelerate wild-type development. Killing all of the bilateral tmc-1 -expressing cells with a laser beam was too challenging to conduct. Thus, as an alternative, we injected into wild type and tmc-1(ok1859) animals a construct containing P tmc-1(3.6k) promoter expressing the membrane-targeted KillerRed [29] , a fluorescent protein that damages/kills cells by releasing reactive oxygen species on illumination. Through manipulating the microscope optics, we localized the illumination on the posterior bulb region of the L1 larvae. When we irradiated the posterior bulb area including SIBD, SIBV, ALA and AVH, wild-type animals did not develop faster on CeMM, indicating that they are not the neurons that attenuate the wild type's development ( Fig. 3b ). However, photodamage to these posterior bulb neurons also did not inhibit development on either CeMM or on the OP50 food ( Fig. 3b ). In contrast, when we irradiated these neurons in tmc-1(ok1859) larvae, the mutant’s growth on CeMM was slowed ( Fig. 3b ); ~23% of the irradiated mutants developed into adults by day 5. Similar to the wild type, removal of these neurons in tmc-1(ok1859) mutants did not inhibit development on OP50. These results argue that some or all of these neurons promote the tmc-1 mutant’s development on the CeMM diet. To assess if the tmc-1 -expressing MC neurons attenuated growth on CeMM, we laser ablated these bilateral cells in wild-type L1 larvae. CeMM-fed operated animals (27%) developed into adults by 5 d.p.h. and most developed into adults by 8 d.p.h. ( Fig. 3c ). To test whether killing any pharyngeal neuron accelerates growth, we ablated one MC and one oppositely located neighbouring pharyngeal NSM neuron, and noted no accelerated development. Thus, removal of both wild-type MC neurons mimics the mutant’s phenotype, suggesting they attenuate growth in the axenic media. Consistent with this, we found that eat-2 mutants developed as fast as tmc-1(rg1003) , and 72% of cha-1 mutants developed into adults by 8 d.p.h. on CeMM ( Fig. 3d ). eat-2 encodes an ionotropic ACh receptor that is expressed in the MC-pharyngeal muscle neuron junction [30] ; thus, an eat-2 null mutation blocks cholinergic transmission from the MC to the pharyngeal muscles [31] ; cha-1 encodes a choline acetyltransferase that synthesizes the neurotransmitter ACh [32] and a cha-1 mutation results in reduced ACh. To test if tmc-1 and eat-2 act in the same pathway, we made an eat-2(ad1113) ; tmc-1(ok1859) double mutant and found that 39% ( n =102) develop into adults at 4 d.p.h. ( Fig. 3e ), and the remainder developed at day 5. This suggests that TMC-1 and EAT-2 might regulate overlapping processes. Together these results imply that TMC-1 stimulates the MC neurons’ cholinergic transmission to the pharyngeal muscles, which attenuates development on CeMM. Since MC ablation mimics the tmc-1 mutant’s phenotype, we asked if TMC-1 changes MC's function. To address this possibility, we ectopically stimulated pharyngeal pumping using serotonin, a process that requires the MC neurons [33] , [34] . We grew wild-type and tmc-1(rg1003) L1 larvae for 2 h on CeMM before the drug test. On 5 mM serotonin application, we found that the wild type had an increased pumping rate compared with the tmc-1 mutants ( Fig. 3f ). These data suggest that when the wild type is fed CeMM, the TMC-1 protein promotes MC’s activity. Since the MC neurons regulate pharyngeal pumping, we asked whether changes in pumping rate and therefore food intake, is correlated with CeMM-regulated development. We measured CeMM-fed wild type and tmc-1(rg1003) L1 larvae pharyngeal contraction rates, but found no differences between the genotypes ( Supplementary Fig. 8 ), indicating the MC’s mode-of-action is subtle. As a control, we found that CeMM-fed eat-2 and eat-2;tmc-1 double mutants both displayed a decreased pumping rate compared with the wild type; however, there was no significant difference between the single and double mutants ( Supplementary Fig. 8 ). Since tmc-1 and eat-2 mutants both develop faster than the wild type, pharyngeal muscle contraction rates are not correlated with regulating larval development on CeMM. TMC-1 has been reported to regulate NaCl sensation through the ASH sensory neurons [15] ; therefore, we asked if these sensory neurons affected developmental rate on CeMM. However, the transgenic expression of TMC-1 in the chemosensory neurons ADL, ADF, AWA and ASH, using the ocr-2 promoter, did not restore a wild-type developmental rate to the tmc-1 mutants ( Fig. 2e ). To test the contributions of these neurons in an alternative way, we hyperpolarized the above sensory neurons in wild-type animals, using a gain-of-function mutant unc-103 voltage-gated K+ channel expressed from the ocr-2 promoter [35] . But unlike crippling the MC neurons, we did not detect accelerated development on CeMM of the unc-103(gf) transgenic line ( Fig. 3c ). TMC-1 slows growth via altering muscle excitability Since we demonstrated that a body wall muscle tmc-1 transgene could partially rescue tmc-1 mutants’ fast growth on CeMM ( Fig. 2e ), we asked if TMC-1 attenuates the development by changing body wall muscles’ physiological state. Since muscle contraction is induced via ACh, we tested the muscles’ physiological state using the ionotropic ACh receptor agonist levamisole (LEV) and the acetylcholinesterase inhibitor aldicarb. Acute LEV application directly induces muscle hypercontraction paralysis [36] , [37] . Whereas because acetylcholinesterase functions to hydrolyse ACh after its release into the synaptic cleft [38] , aldicarb indirectly induce hypercontraction paralysis through build-up of an unhydrolysed neurotransmitter. We picked L4 larval hermaphrodites from NGM OP50 plates, and grew them on CeMM plates for 18–20 h before the drug test. We found that the LEV EC50 for the wild-type and tmc-1(rg1003) mutant are 4.76 and 15.68 μM, respectively ( Fig. 4a ). Since wild-type body wall muscles are more sensitive to LEV, TMC-1 may promote body wall muscle depolarization. In addition, we observed that when hermaphrodites developed into adults on NGM OP50, they displayed similar sensitivity to LEV, despite their genotype (EC50: N2=6.8 μM, tmc-1(rg1003) mutant=5.3 μM; Fig. 4b ). Similarly, we found that the wild type was more sensitive to aldicarb if L4 larvae grew on CeMM for 20 h before the drug test ( Fig. 4c ), but not when they were fed OP50 ( Fig. 4d ). These findings suggest that TMC-1 promotes body wall muscle excitability, but only in the altered growth environment of CeMM. 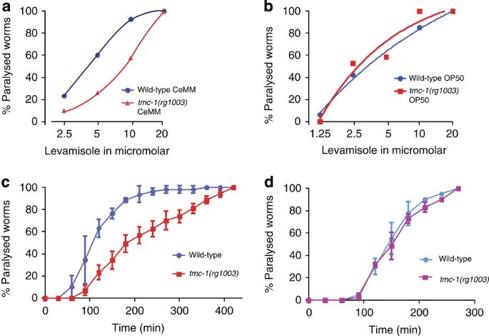Figure 4: TMC-1 attenuates development through changing body wall muscles’ excitability. (a) The response of the worms’ body wall muscles to different concentrations of the ACh agonist LEV. L4 larval hermaphrodites were picked from NGM OP50 plates and grown on CeMM plates for 18–20 h before the drug test. We observed worms in the LEV solution for 5 min. Animals that failed to move during the observation period were scored as paralyzed. More than 30 worms were assayed for each concentration. The EC50 for wild type and thetmc-1(rg1003)mutant is 4.76 and 15.68 μM, respectively. (b) The response of the worm’s body wall muscles to different concentrations of the ACh agonist LEV. L4 larval hermaphrodites were picked from NGM OP50 plates, and grown in NGM OP50 plates for 18–20 h before the drug test. More than 30 worms were assayed for each concentration. The EC50 for wild type and thetmc-1(rg1003)mutant is 6.8 and 5.3 μM, respectively. (c) The response of the worms’ body wall muscles to aldicarb. The experiments were conducted on nematode growth media (NGM) plates containing 1 mM aldicarb. L4 larval hermaphrodites were picked from NGM OP50 plates and grown on CeMM plates for 20 h before the drug test. Each data point represents the mean percentage of animals paralysed by aldicarb. Animals were scored every 30 min for the three drug-soaked plates, totalling a minimum of 50 animals. Error bars represent s.d. (d) The response of the worms’ body wall muscle to aldicarb. L4 larval hermaphrodites were picked from NGM OP50 plates and grown in NGM OP50 plates for 20 h before the drug test. Each data point represents the mean percentage of animals paralysed by aldicarb. Animals were scored every 30 min for two trials, totalling a minimum of 40 animals. Error bars represent s.d. Figure 4: TMC-1 attenuates development through changing body wall muscles’ excitability. ( a ) The response of the worms’ body wall muscles to different concentrations of the ACh agonist LEV. L4 larval hermaphrodites were picked from NGM OP50 plates and grown on CeMM plates for 18–20 h before the drug test. We observed worms in the LEV solution for 5 min. Animals that failed to move during the observation period were scored as paralyzed. More than 30 worms were assayed for each concentration. The EC50 for wild type and the tmc-1(rg1003) mutant is 4.76 and 15.68 μM, respectively. ( b ) The response of the worm’s body wall muscles to different concentrations of the ACh agonist LEV. L4 larval hermaphrodites were picked from NGM OP50 plates, and grown in NGM OP50 plates for 18–20 h before the drug test. More than 30 worms were assayed for each concentration. The EC50 for wild type and the tmc-1(rg1003) mutant is 6.8 and 5.3 μM, respectively. ( c ) The response of the worms’ body wall muscles to aldicarb. The experiments were conducted on nematode growth media (NGM) plates containing 1 mM aldicarb. L4 larval hermaphrodites were picked from NGM OP50 plates and grown on CeMM plates for 20 h before the drug test. Each data point represents the mean percentage of animals paralysed by aldicarb. Animals were scored every 30 min for the three drug-soaked plates, totalling a minimum of 50 animals. Error bars represent s.d. ( d ) The response of the worms’ body wall muscle to aldicarb. L4 larval hermaphrodites were picked from NGM OP50 plates and grown in NGM OP50 plates for 20 h before the drug test. Each data point represents the mean percentage of animals paralysed by aldicarb. Animals were scored every 30 min for two trials, totalling a minimum of 40 animals. Error bars represent s.d. Full size image The GABA A agonist muscimol relaxes the body wall muscles, also causing C. elegans paralysis [39] . For the muscimol assay, L4 larva hermaphrodites were picked from NGM OP50 plates, and grown on CeMM plates for 18–20 h before the drug test. The EC50 for the wild type and tmc-1(rg1003) mutant is 2.555 and 2.661, respectively ( Supplementary Fig. 9 ). This finding suggests that TMC-1 does not play an obvious role for body wall muscle GABAnergic inhibition. Published work has reported that the microRNA mir-1 , neurexin and neuroligin promote retrograde signalling between the body wall muscles and the ventral cord neurons [40] . Since TMC-1 is also expressed in the body wall muscles, we asked if reducing mir-1 also accelerates development on CeMM. We assayed three mir-1 mutant alleles. The n1401 and n4102 mutants had a similar developmental rate as the wild type ( Supplementary Fig. 10 ). But after 10 days of growing on CeMM, we measured a small, but statistically higher percentage of mir-1(gk276) adults, compared with the wild type and the n4101 and n4102 mutants (N2, 51% adults; mir-1(gk276) , 70% adults; P =0.03). Although mir-1 mutants display less sensitivity to LEV and aldicarb in standard food conditions [41] , we do not think mir-1 ’s role on retrograde signalling and muscle function has a major effect on slowing growth on CeMM media. tmc-1 mutants show increased ATP and O 2 usage We hypothesize that the tmc-1 larvae can metabolize the constituents of CeMM better than the wild type, allowing the mutant to develop faster. Since developing animals require energy from their food to support their development, we asked if the fast developing tmc-1 mutant larvae have higher levels of ATP [42] . We determined the amount of ATP in 20,000 L1 wild-type and tmc-1(rg1003) larvae were either kept in M9 or CeMM-fed for 2 h. After the feeding/incubation period, we homogenized the worms and measured their ATP content using a Luciferase assay. We found that in M9, tmc-1 and wild-type larvae had similar amounts of ATP, but after 2 h of CeMM feeding, the wild type contained less ATP relative to the tmc-1 animals ( Fig. 5a ). The increased ATP could supply energy for tmc-1 mutants to support fast development on CeMM. 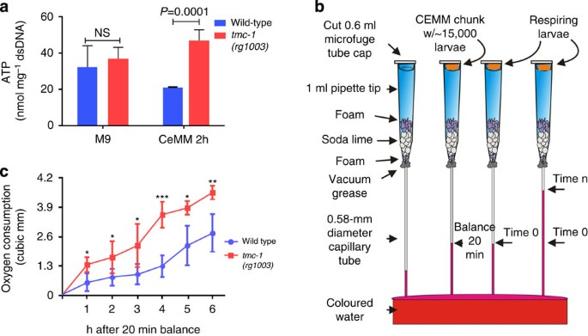Figure 5:tmc-1mutant larvae showed increased ATP levels and O2consumption for supporting fast development. (a) ATP concentration after 2 h culture of N2 ortmc-1(rg1003)in CeMM. (n=2 trials; mean±s.d., Student’st-test). (b) Cartoon of the lab-made respirometer. Adapted from ref.43. (c)tmc-1(rg1003)mutant larvae showed increased oxygen consumption. Oxygen consumption was measured in CeMM with lab-made respirometers (n=4 trials; mean±s.d., Student’st-test). Figure 5: tmc-1 mutant larvae showed increased ATP levels and O 2 consumption for supporting fast development. ( a ) ATP concentration after 2 h culture of N2 or tmc-1(rg1003) in CeMM. ( n =2 trials; mean±s.d., Student’s t -test). ( b ) Cartoon of the lab-made respirometer. Adapted from ref. 43 . ( c ) tmc-1(rg1003) mutant larvae showed increased oxygen consumption. Oxygen consumption was measured in CeMM with lab-made respirometers ( n =4 trials; mean±s.d., Student’s t -test). Full size image The increased ATP levels should be correlated to increased metabolism and oxygen consumption. Oxygen consumption was measured in animals fed on CeMM with lab-made respirometers ( Fig. 5b ) [43] . We found that tmc-1(rg1003) mutant larvae showed increased oxygen consumption compared with the wild type after 2 h growth on CeMM ( Fig. 5c ). These data imply that tmc-1(rg1003) larvae can utilize the CeMM food for energy more efficiently than the wild type. We also asked if the tmc-1 mutant L1 larva initially catabolize their embryonic-derived fat reserves better than the wild type. However, staining with Nile Red [44] , we found that this was not the case. Before and after growth on CeMM or OP50 for 2 h, the wild type and tmc-1 L1 larvae still had similar intestinal fat levels. Not surprisingly, when fed OP50 for 2 h, both types of animals had higher fat levels compared with CeMM-fed worms ( Supplementary Fig. 11 ). We favour the simple explanation that the tmc-1 mutants are better at using the CeMM constituents for catabolic and anabolic processes, rather than solely relying on the fat stores they acquired at hatching. However, we do not rule out the possibility that after the tmc-1 mutants ingest CeMM, they convert some of the CeMM constituents into intermediate macro molecules (lipids, proteins and long-chain sugars), which they subsequently catabolize by consuming O 2 to generate ATP. Mutant tmc-1 -induced growth requires insulin signalling The insulin pathway is critical for development, lifespan, stress resistance and metabolism [45] . Therefore, we asked if the tmc-1 mutants’ fast growth on CeMM depends on this pathway. To address this question, we assayed the development of several insulin pathway-related mutants on CeMM. We found that under permissive temperatures, the growth of the daf-2 insulin receptor temperature sensitive mutants, ( m41 and e1368 ), on CeMM was slower than the wild type ( Fig. 6a ). Although DAF-2 negatively regulates the FOXO transcription factor/DAF-16, we found that mutations in either gene further attenuated growth on CeMM. When daf-16(mu86) animals were grown on CeMM, 4% ( n =80) developed into adults at 6 d.p.h., 8% developed into adults at 8 d.p.h., while only 29% developed into adults at 14 d.p.h. ( Fig. 6a ). Thus, both molecules are required for animals to develop on CeMM. 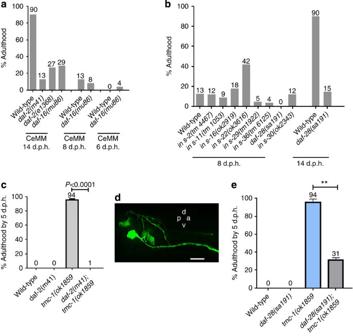Figure 6: The accelerated development oftmc-1mutants require insulin pathway components. (a) Growth rate ofdaf-2anddaf-16(n=30–100; one trial). (b) Growth rate ofdaf-2(m41);tmc-1(ok1859)double mutants (50–70 worms/trial; three trials mean±s.d., Student’st-test). (c) Growth rate of several insulin pathway mutants (n=40–100; one trial). (d) Fluorescence image ofdaf-28::YFP (e) Growth rate ofdaf-28(sa191);tmc-1(ok1859)double mutants (n=60–80 worms per trial; two trials; mean±s.d., Student’st-test). Data were presented as mean±s.d. (*P<0.05, **P<0.01, ***P<0.001) A, anterior; D, dorsal; P, posterior; V, ventral. White arrows indicate expression in specified neurons or tissues. Scale bars, 10 μm. Figure 6: The accelerated development of tmc-1 mutants require insulin pathway components. ( a ) Growth rate of daf-2 and daf-16 ( n =30–100; one trial). ( b ) Growth rate of daf-2(m41);tmc-1(ok1859) double mutants (50–70 worms/trial; three trials mean±s.d., Student’s t -test). ( c ) Growth rate of several insulin pathway mutants ( n =40–100; one trial). ( d ) Fluorescence image of daf-28 ::YFP ( e ) Growth rate of daf-28(sa191);tmc-1(ok1859) double mutants ( n =60–80 worms per trial; two trials; mean±s.d., Student’s t -test). Data were presented as mean±s.d. (* P <0.05, ** P <0.01, *** P <0.001) A, anterior; D, dorsal; P, posterior; V, ventral. White arrows indicate expression in specified neurons or tissues. Scale bars, 10 μm. Full size image We next checked if a daf-2 mutation can slow the larval development of the tmc-1 mutant. The daf-2(m41);tmc-1(ok1859) double mutant had no obvious developmental defect when grown on OP50, but the mutant grew slower compared with the tmc-1 single mutant on CeMM ( Fig. 6b ), suggesting that the tmc-1 fast growth depends on the insulin pathway. Since the insulin pathway is involved, we asked which insulin-like peptide can regulate CeMM-mediated development. We determined the growth rate for several insulin-like peptide mutants and found that most of them had a similar growth rate on CeMM as N2. However, ins-22 mutants showed a faster development (at day 8, 42% grew to adults; Fig. 6c ); and the daf-28 mutant developed slower (15%, by 14 d.p.h. ; Fig. 6c ). This suggests that insulin-like peptide DAF-28 might be candidate insulin-like ligand for CeMM growth. daf-28 is expressed in several head neurons including ASI [46] ( Fig. 6d ), which is known to play a critical role in calorie restriction dependent longevity, and in a developmental decision to survive a nutritionally harsh environment [20] . However, we did not detect an expression overlap between the insulin-expressing neurons and the tmc-1 -expressing neurons. The insulin ligand and TMC-1-expressing neurons have processes in or near the C. elegans nerve ring, suggesting that diffusion over ~100–200 μm could be sufficient for their communication [47] . We asked if daf-28 plays a similar role as daf-2 in suppressing tmc-1 mutants’ fast growth on CeMM. We made the daf-28(sa191);tmc-1(ok1859) double mutant. Similar to the daf-2(m41) mutation, the daf-28 mutation also slowed down the growth rate of CeMM-fed tmc-1 worms ( Fig. 6e ). However, the extent of suppression is less severe compared with the daf-2(m41) mutation ( Fig. 6b ). This finding suggests that DAF-28 might be one of many insulin receptor ligands required for CeMM growth. Mutant tmc-1 promotes male mating behaviour on CeMM To establish a population in novel nutrient environments, an organism must also sexually reproduce in the locale. Since TMC-1 restrains the larval development on CeMM, we asked if it might also affect sexual reproduction after development. Therefore, we examined the sexual potency of tmc-1(rg1003) males on CeMM. The tmc-1 mutation does not affect male mating behaviour under standard conditions ( Fig. 7a ). When males were raised and subsequently allowed unlimited mating on OP50, wild-type and tmc-1 mutant males mated with similar potency ( Fig. 7a ). In contrast, when wild-type males were raised on CeMM media, none ( n =30) were able to sire cross-progeny under unlimited mating conditions ( Fig. 7a ). However, 43% of the tmc-1 mutants ( n =30) were able to sire cross-progeny ( Fig. 7a ). To determine if the CeMM media components were not inhibiting mating behaviour through non-specific means, we first fed wild-type and tmc-1 mutant males OP50 from L1 larval stage to adulthood, and then conducted the unlimited mating assay on CeMM. We reasoned that if CeMM irritated the males, then the mating potency of OP50-fed males should be the same as CeMM-fed males. We found that the mating potency for both OP50-fed males were much higher than CeMM-fed males, indicating that this was not the case. However, tmc-1 males were still more potent than wild-type males ( Fig. 7a ). Thus, regardless if the male developed on CeMM or OP50 food, mutating tmc-1 can increase sexual fitness on the CeMM media. We then asked if similar sets of neurons that use tmc-1 to regulate larval development, also regulate mating behaviour. We tested the mating potency of OP50-fed tmc-1(rg1003) males containing the full-length P unc-17(10k) : tmc-1 cDNA construct and found that their mating potency reverted back to the low wild-type-like level ( Fig. 7a ). These data demonstrate that similar neurons might regulate both development and reproduction. 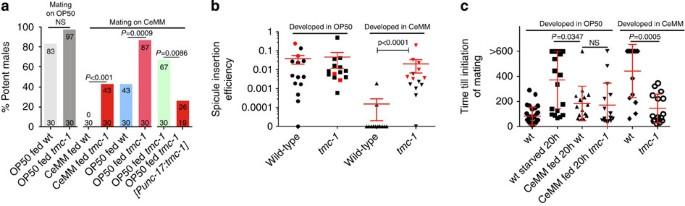Figure 7: Mutanttmc-1promotes mating behaviour. (a)tmc-1(rg1003)mutants had higher male mating potency than wild type (wt) on CeMM. Strain expressedtmc-1cDNA using the full-lengthunc-17promoter (10k) rescuedtmc-1(rg1003)mating potency on CeMM. 1-day-old males were grown in NGME. coliOP50 plates or CeMM plates from the L1 larval stage, before being used in the CeMM mating assays (nis listed in the bottom of the columns, Fisher’s exact test). (b)tmc-1(rg1003)mutants had higher male mating efficiency (ESI) than wild type on CeMM, when males were grown on CeMM plates from L1 larvae (red represent successful insertion,n=14, mean±s.d., Mann–Whitney non-parametric test). (c) Mean time till initiation of mating in bacterial food source (wild type ortmc-1(rg1003)mutant were used,n=15, mean±s.d., Mann–Whitney non-parametric test). Figure 7: Mutant tmc-1 promotes mating behaviour. ( a ) tmc-1(rg1003) mutants had higher male mating potency than wild type (wt) on CeMM. Strain expressed tmc-1 cDNA using the full-length unc-17 promoter (10k) rescued tmc-1(rg1003) mating potency on CeMM. 1-day-old males were grown in NGM E. coli OP50 plates or CeMM plates from the L1 larval stage, before being used in the CeMM mating assays ( n is listed in the bottom of the columns, Fisher’s exact test). ( b ) tmc-1(rg1003) mutants had higher male mating efficiency (ESI) than wild type on CeMM, when males were grown on CeMM plates from L1 larvae (red represent successful insertion, n =14, mean±s.d., Mann–Whitney non-parametric test). ( c ) Mean time till initiation of mating in bacterial food source (wild type or tmc-1(rg1003) mutant were used, n =15, mean±s.d., Mann–Whitney non-parametric test). Full size image To determine why the tmc-1 mutants were more potent on CeMM, we used a mating observation assay, the spicule insertion efficiency ( E SI ). The assay combines in one metric how fast males sustain, reattempt and complete insertion into the hermaphrodite vulva of their copulatory organs, the spicules [48] . When males were developed in OP50 and their various copulatory behaviours were observed on CeMM, we did not detect any difference in spicule insertion efficiency between wild type and mutant ( Fig. 7b ). In contrast, when the males developed on CeMM, we found that tmc-1 mutants had a higher spicule insertion frequency than the wild type ( Fig. 7b ), and similar to males that were raised on OP50. This indicates that the development in CeMM (and not an acute exposure to CeMM) affected the motor capabilities of wild-type animals. Since nutrient availability affects not only the development but also the mating ability [35] , we hypothesized that an extended exposure to CeMM media might induce a starvation response in wild-type males, but not in tmc-1 males. This could reduce the wild-type male’s ability to initiate mating behaviour. To address this possibility, we raised males on CeMM or OP50, and then fed the L4 males CeMM for 20 additional hours. We then put the males outside an OP50 bacterial lawn that contained 10 hermaphrodites and measured (in a 10-min observation period) the duration required for the males to initiate mating after they entered the lawn ( Fig. 7c ). We hypothesized that if the males were starving in CeMM, then when they crossed into the bacterial lawn, they would spend part of the observation period eating, rather than copulating. As a control, we starved OP50-fed wild-type males for 20 h, and found that OP50-raised/CeMM-fed wild-type males initiated mating significantly faster than OP50-raised/starved wild-type males ( Fig. 7c ). Thus, CeMM feeding does not elicit the same effect as starvation. We then compared OP50-fed wild-type and OP50-fed tmc-1 mutant males and found no differences in the time required to initiate mating ( Fig. 7c ). But when we conducted this assay on wild-type and tmc-1 males that were raised in CeMM throughout the development, the tmc-1 males behaved like the OP50-fed males, and wild-type males behaved like the OP50-raised/20 h-starved males ( Fig. 7c ). Taken together, these data demonstrate that TMC-1 has a developmental effect, (and to a lesser extent, an acute effect) on repressing both appetitive (mating drive) and consumatory (spicule insertion) sexual behaviours on CeMM. Mutations in insulin and serotonin pathway genes have been shown to perturb development and mating, in a bacterial food source [35] , [49] , whereas our results showed that the tmc-1 mutation displayed an opposite effect, which accelerates larval development and male mating on CeMM. The worm has provided insights on how different dietary nutrients affect life history traits, such as developmental rate, reproduction and lifespan. For example, when fed with Comamonas bacteria, wild-type C. elegans develop and age faster than when fed the standard laboratory E. coli OP50 (refs 3 , 50 ). Also, mutants in the nuclear hormone receptor gene nhr-114 are sterile when fed with E. coli OP50, but not the strain HT115. The failure to thrive on certain bacteria can be rescued by tryptophan supplementation [51] . Finally, the alh-6 mutant exhibit a diet-specific reduction in lifespan when fed with E. coli OP50 (refs 52 , 53 ). These studies show how different bacterial food modifies worm growth and aging. CeMM can also be used to study worm growth and aging, since the media removes the complications of bacterial secondary metabolites. Slow development and poor reproduction are indicators of nutritional stress [54] . A commonly studied stress is dietary restriction, which can slow down/arrest development and reduce sexual behaviour [12] , [55] . In contrast to dietary restriction, where nutrients are limited, the synthetic CeMM food contains the basic nutrients in excess. However, since others have reported that C. elegans superficially responds to CeMM similarly to dietary restriction [12] , the stress that the animal experiences might be related to the suboptimal presentation of the nutrients and the low efficiency of nutrient utilization. Although the population growth is slower in CeMM compared with a bacterial diet [10] , the population will eventually grow to high density. Therefore, the rate of nutrient utilization might be the limiting factor in developing on CeMM. Our work suggests that the worm has the ability to better utilize the media. We hypothesize that C. elegans uses the TMC-1 molecule as part of its stress sensing system to delay the rate of biological processes, such as development and reproduction, until the animal finds more familiar food. When N2 larvae are fed CeMM, they require up to 2 weeks to sexually mature. In contrast, tmc-1 mutations relax growth restriction and allow the animals to metabolize CeMM fuel. Consequently, the mutants develop into adults by 5 days, and males display successful sexual behaviours. Although CeMM-fed tmc-1 mutants develop faster, they are not optimized in their physiology. As adults, the CeMM-fed tmc-1 mutants resemble their slow developing wild-type counterparts; they are still thin and have a dietary restricted-like appearance. We hypothesize that unfamiliar food (such as CeMM) dampens growth and behaviours in wild type through mechanisms that respond to mild stress, but the tmc-1 mutants are deficient in these processes. C. elegans TMC-1 is reported to be a sodium-gated ion channel. It facilitates the ASH sensory neurons in detecting stressful levels of external sodium and directing an aversive behavioural reflex [15] . In our work, we found that TMC-1 promotes both MC and body wall muscles’ excitability, as a downstream response to perceived foreign food. The increased excitability might be via sodium influx, which would be consistent with experiments demonstrating TMC-1-mediated sodium conduction [15] . However, we found that increased environmental sodium has no obvious effect on development for both CeMM-fed wild type and tmc-1(rg1003) mutants. These findings suggest that TMC-1 might have other functions to regulate the cell’s physiology, in addition to aversive environmental sodium sensation. We propose that TMC-1 indirectly or directly transduce or amplify mild internal stress signals in neurons and muscles. Depending on the type of stress and the responding neural muscular circuit, the resulting increased cell excitability could subsequently promote secretion signals, which alter worm development and behaviour. However, we do not rule out the possibility that TMC-1 might also have receptor/sensor-like properties. The mammalian homologue TMC-1 is linked to deafness [16] , [17] , [18] , and it is reported to be a mechanotransduction channel component of inner ear hair cells [16] , [56] . Thus, TMC proteins, including but not limited to the mammalian TMC-1, could function as ionotropic sensory receptors; although they might be regulated by ligands in addition to sodium [15] . In our CeMM paradigm, TMC-1 shows a context-dependent function for both development and male mating behaviour. On OP50 food, tmc-1 mutants are wild type for development and male mating potency, but display adapted traits for increased growth rate and male mating potency on CeMM food. As environmental challenges are linked to organismal evolution, genes like TMC-1 might be used for determining when an animal should acclimate to an unfamiliar environment. Genetic outcrossing is favoured in populations of C. elegans subjected to hostile conditions, such as mutagenic environments and pathogen bacteria [57] . However, these same conditions elicit escape responses and thus acutely reduce male sexual libido and copulation execution (our unpublished observations). Our findings that tmc-1 mutants display increased male mating potency implies that natural down-regulation of TMC-1 might be required to promote outcrossing in non-familiar conditions. In CeMM, the sites of action for TMC-1 in regulating developmental rate include the cholinergic pharyngeal MC motor neurons and body wall muscles. MC ablation in wild-type larvae is sufficient to accelerate their growth in CeMM, indicating that they are involved in how the animal couples mechanical nutrient intake with cellular growth rate. Under standard bacterial diet conditions, the MCs regulate pharyngeal pumping rate through secreting ACh to the pharyngeal muscles [4] , [34] , [58] . Our results show that ablation of the MC neurons in the wild type accelerates the developmental rate, suggesting that TMC-1 promotes developmental retardation partly through these neurons. We also report additional genetic data to support the MC neurons’ role on regulating growth on CeMM. eat-2 and cha-1 mutants develop faster on the synthetic media. eat-2 encodes an ACh receptor expressed in the MC-pharyngeal neuromuscular junction and cha-1 encodes an ACh biosynthetic enzyme. Thus, we speculate that tmc-1 mutants promote C. elegans growth through subtly reducing MC neurons’ ACh secretion to the pharyngeal muscles. We also showed that tph-1 and ser-7 mutations promote growth on CeMM and eat-4 mutations promote a fast growth rate analogous to tmc-1 and eat-2 mutations ( Fig. 3d and Supplementary Fig. 12 ). These genes are expressed broadly, but also have a presence in the pharyngeal nervous system. Under standard conditions, mutations in these genes disrupt pumping rhythmicity. tph-1 is expressed in the NSM pharyngeal neurons and encodes tryptophan hydroxylase, which catalyses the first step in serotonin biosynthesis [59] . ser-7 encodes a type 7 serotonin receptor, and is expressed in pharyngeal neurons including the MC neurons [34] , [60] , [61] , and SER-7 is the major serotonin receptor to stimulate MC. eat-4 encodes a vesicular glutamate transporter and is expressed in the pharyngeal M3 neurons [62] , [63] . Taken together, other pharyngeal neurons, in addition to MC, could contribute to attenuating growth rate on CeMM. Because the tmc-1 mutations do not obviously affect pharyngeal muscle contractions, we speculate that the pharynx might play an additional accessory signalling role in regulating how the animal coordinates development and catabolism. The pharynx has been reported to express growth factors such as LIN-3 (EGF), LET-756 (fibroblast growth factor-like ligand) and insulin-like peptides; thus, this tissue might have regulatory endocrine functions in addition to being a contractile organ [64] , [65] , [66] . In addition to identifying molecules that restrain development in CeMM, we also showed that DAF-2 signalling is required for growing in CeMM. The DAF-28 insulin-like peptide is likely one of many ligands that the CeMM-fed animal requires to stimulate the DAF-2 receptor. The TMC-1 proteins are broadly expressed and we postulate that TMC-1 might negatively regulate some of these cells (such as SIB, ALA and AVH) from directly or indirectly promoting developmental and behavioural relevant insulin-like peptide secretion. In conclusion, this study demonstrates that single-allele changes can direct both development and reproductive behaviour, so that evolving animals can adapt to- and sexually reproduce in changing environmental circumstances [57] , [67] . Strains and culture Strains were grown at 20 °C on CeMM 1.7% agarose plates or NGM plates with OP50 bacteria [10] . tmc-1(rg1003) mutant was identified in this study. tmc-1(ok1859) was used in experiments where the deletion allowed straightforward genotype identification using the PCR-based size polymorphism. A complete list of strains is given in Supplementary Table 1 . CeMM preparation 2 × CeMM stock media was prepared with 54 chemicals, including vitamins and growth factor solutions, salt solutions, amino acids, nucleic acid substituents, described in Supplementary Table 2 . The above chemical solutions were mixed together and reduced glutathione, choline, myoinositol, cytochrome C, glucose, β-sitosterol, streptomycin (200 mg l −1 ), and kanamycin (40 mg l −1 ) were subsequently added to the mixed solution. The pH of the solution was adjusted to 5.2 using 10% (w/v) KOH. The media was filter sterilized using a Corning 0.2 μm filter system. We found that C. elegans N2 developed even slower if the solution had a pH lower or greater than 5.2. The media was diluted to 1 × by adding an equal volume of molten 3.4% agarose solution. Petri dishes of 3.5 cm diameter contained 5 ml of CeMM-agarose. Hermaphrodites were age-assessed based on the developmental stage of the vulva, while males were age-assessed based on the developmental stage of their proctodeum. Dauers (3 and 4%) were found on CeMM plate at 8 and 10 d.p.h., for daf-2 ( n =75) and daf-28 ( n =50), respectively. tmc-1 identification The tmc-1(rg1003) mutant was identified by EMS-mutagenized N2 hermaphrodites. In the second generation, gravid hermaphrodites were treated with an alkaline hypochlorite solution to release the eggs from their uterus. The eggs were kept on NGM plates without bacteria and arrested L1 larvae were then transferred to CeMM plates. The fastest developing animals that were also grossly normal in development and behaviour were then isolated. Outcrossing experiments demonstrated that fast growth on CeMM, caused by the rg1003 allele, is inherited as a single-locus recessive trait. Using classical two-point mapping, we mapped rg1003 mutation to the left end of X chromosome. Then, using Illumina next-generation sequencing followed by sequence data analysis with MAQGene [68] , Sanger resequencing and a complementation test with mutant line tmc-1(ok1859) , we mapped the rg1003 mutation to tmc-1 . Molecular biology and generation of transgenic lines An 8.4-kb fragment containing 3.6 kb upstream of the start site of tmc-1(T13G4.3) , 4.8 kb of exon 1 to partial exon 3 was PCR-amplified from N2 genomic DNA. The sequences of the primers used are shown below: Attb1T13G4F1: 5′- ggggacaagtttgtacaaaaaagcaggctTTTGAATGTTGGCTCCGGTGGTCC -3′ Attb2T13G4R1: 5′- ggggaccactttgtacaagaaagctgggtCCTTGTTGATGAATGCATCGGTTTC -3′ The PCR primers contained Gateway ATTB sites, which allowed the 8.4-kb PCR products to be recombined, using BP clonase (Invitrogen), into the Gateway entry vector pDG15, to generate pLZ1. pLZ1 was recombined with the YFP destination vector pGW322YFP, using LR clonase (Invitrogen) to make pLZ2. The 18.4-kb tmc-1 genomic region from 3.6 kb upstream of the start site to 1.2 kb after the stop codon was amplified through three overlapping genomic regions using 5′- TTTGAATGTTGGCTCCGGTGGTCC -3′ and 5′- CCTTGTTGATGAATGCATCGGTTTC -3′; 5′- TTTGAATGTTGGCTCCGGTGGTCC -3′ and 5′- CTCTATGACATTCTCTACGCGT -3′; 5′- AAAATCCCAAGTGCAAGACG -3′ and 5′- GTTGAACAATGGGGTGCAATACTGA -3′ primers. The tmc-1 cDNA was amplified with 5′- TACAAAGTGGTGATCATGCAGGAAGCGGCAAGGAGAG -3′ and 5′- CTGTTGGGGGATCCTTCAATCAATTTGCCGCGGAGAGT -3′ primers, from the cDNA clone yk1488c10 (a gift from Professor Yuji Kohara). The plasmid pYL30, which contained the ATTB Gateway destination cassette A, SL2 trans -splice site and green fluorescent protein, was PCR-linearized with 5′- AGGATCCCCCAACAGAGTTGTTGA -3′ and 5′- GATCACCACTTTGTACAAGAAAGC -3′ primers. The tmc-1 cDNA was inserted between the linearized ends of pYL30, in a region after the Gateway destination cassette A, but before the SL2-green fluorescent protein site, using the In-Fusion HD EcoDry Cloning Kit (Clontech), to make the plasmid pLZ8. The primers 5′- ggggacaagtttgtacaaaaaagcaggctTGCAGACTTTTCCCCAAACTAGC -3′ and 5′- ggggaccactttgtacaagaaagctgggtGACGGGCACGTTGAAGCCCAACT -3′ were used to PCR amplify an ~3.7 kb upstream region of the unc-17 vesicular ACh transporter gene; this region drives the expression in the cholinergic head neurons. The primers 5′- ggggacaagtttgtacaaaaaagcaggctGTGTATGGTGGTGGAGCATTCGACAT -3′ and 5′- ggggaccactttgtacaagaaagctgggtGACGGGCACGTTGAAGCCCAACT -3′ were used to PCR amplify an ~10 kb upstream region of the unc-17 vesicular ACh transporter gene, which promotes the expression in all cholinergic neurons. The reverse primer mutates the ATG of the first exon to TTG. The primers also contained Gateway ATTB sites, which allowed the PCR products to be recombined, using BP clonase (Invitrogen, CA) into the Gateway destination vector pDG15, to generate pLR159 (3.7 kb upstream) and pBL228 (10 kb upstream). The 3.5-kb upstream region of lev-11 in pLR22 and the 3.7 and 10 kb upstream region of unc-17 in pLR159 and pBL228, respectively, were recombined into pLZ8 using LR clonase (Invitrogen) to make the plasmids pLZ9, pLZ10 and pLZ11. A 3.6-kb fragment upstream of ATG of tmc-1 was PCR-amplified from N2 genomic DNA. The sequences of the primers used are shown below: Attb1T13G4F1: 5′- ggggacaagtttgtacaaaaaagcaggctTTTGAATGTTGGCTCCGGTGGTCC -3′ Attb2T13G4R5: 5′- GgggaccactttgtacaagaaagctgggtTTTGATAGTCGTCGGAGCAAGAGT -3′ The 3.6-kb upstream region was recombined into the Gateway entry vector pDG15, using BP clonase (Invitrogen), to generate pLZ12. Then, pLZ12 was recombined with pLR305, which contained the Gateway destination cassette C.1, GCaMP6, SL2 and DsRed, using LR clonase (Invitrogen) to make pLR307, or was recombined with pCJ45, which contained the Gateway destination cassette C.1and membrane-targeted KillerRed (cloned from pKillerRed-mem vector Cat.#FP966, Evrogen, Russia) to generate pLZ15. A complete list of transgenic strains is given in Supplementary Table 3 . Laser ablation The operations were conducted using a Spectra-Physics VSL-337ND-S Nitrogen Laser (Mountain View, CA) attached to an Olympus BX51 microscope. MC or NSM neurons were identified by cell position using DIC optics. Cells were killed at L1 larval stage after arrested starved L1 larvae were cultured in NGM E. coli OP50 plates for 1 h, which helped give better visual definition to the target cells under DIC optics. Ablated and mock-ablated L1 worms were operated on 2.5% agar pads containing 7.5 mM NaN 3 . Operated animals were kept on CeMM plates at 20 °C, and their growth rates were observed during the following eight days. Photoablation New hatched L1 larvae were illuminated on 8% agar pads containing Polybead polystyrene 0.1 μm microspheres (Polysciences Inc., PA) [69] . Transgenic worms, containing the KillerRed protein, were mounted on an Olympus BX51 microscope. Through pulling out the field iris diaphragm knob, illumination region was specified, using × 100 magnification objectives, over the areas of the SIBD, SIBV, ALA and AVH neurons. The area was illuminated with 561 nM epi-fluorescence light and the emitted red fluorescence was monitored through a 607-nM filter. The cells were illuminated until they no longer fluoresced, which was about 2 min. Animals were kept on CeMM plates at 20 °C, and their growth rates were observed in the following 8 days. After the eighth day, animals were remounted to determine if the target illuminated neurons were killed or were still intact. Pharyngeal pumping rate assays Pharyngeal pumping rates (pumps per min) were measured by counting the contraction of the pharyngeal bulb over a 30-s period. Worm pumping behaviour was digitally recorded at 30 frames per second, using an Olympus BX51 microscope equipped with a long working distance × 60 objective and a Hamamatsu ImagEM digital camera. For CeMM-induced pumping rate determination, L1 larvae were transferred to a CeMM chunk. Pumping behaviours were recorded after 2 h of CeMM growth. Image stacks were slowed down and reviewed using HCImage software (Hamamatsu). Calcium imaging The genetically encoded calcium sensor GCaMP6 (ref. 25 ) was used to visualize calcium transients in MC, SIBD, SIBV, ALA and AVH neurons. We found that the CeMM media autofluoresces under the 480-nm excitation light needed to visualize G-CaMP fluorescence. To work around this problem, we imaged the animals before they were fed CeMM; then after a period of growth, we removed the animals from CeMM and immediately imaged them again. The red fluorescent protein DsRed was expressed in the same set of cells as GCaMP as an internal control. The GCaMP and DsRed fluorescence signals were recorded simultaneously using a Dual View Simultaneous Image splitter (Photometrics, AZ) and a Hamamatsu ImagEM Electron multiplier (EM) CCD camera. The Ca 2+ data were analysed using the Hamamatsu SimplePCI (version 6.6.0.0) software and Microsoft Excel, as described [70] . For both the wild-type and tmc-1(ok1859) mutants, individual starved L1 larvae were first mounted on a 2.5% agarose pad with coverslip and allowed to crawl freely. Using a long working distance × 40 objective, animals were illuminated using an excitation filter set that allowed simultaneous transmission of 480 and 570 nm light, and an image splitter fitted with an emission filter set that allowed transmission of 520 and 630 nm light. Crawling animals were illuminated and recorded (30 frames per second) for 30 s to minimize bleaching. Animals were then put on CeMM plates for 2 h. The fed animals were then remounted on a 2.5% agarose pad with a coverslip, and the moving animals were re-illuminated/recorded using the identical camera exposure settings. To analyse the data, the 30-s recordings were reviewed to find 5 to 10 frames where the cells of interest were in focus. Regions of interests were placed over the cells of interest in both green and red channels in those frames. Average pixel intensities in the regions of interests were calculated for both background and the cells of interest in both green and red channels. Only animals where the average pixel intensity in the red channel did not change after feeding were further analysed; reduction in the red channel after feeding indicated photo-bleaching during the first recording. The background-subtracted steady-state green over red ratio was calculated for the 5 to 10 frames and then averaged. For each cell type of interest, the fold change of the green/red ratio for CeMM- or OP50-fed L1 animals relative to starved L1 animals was then calculated. If there was no change between CeMM-fed animals and the starved animals, then the ratio would be 1. Ratios >1 indicate higher calcium transients in CeMM-exposed animals; ratios <1 indicate lower calcium transients. ATP assay L1 larvae (20,000) that were either kept in M9 or fed for 2 h with CeMM were collected, frozen and thawed three times. The worms were homogenized using the Bullet Blender (Next Advance) and the supernatant was collected and measured using an ATP Determination Kit (Life Technology, NY) and were normalized to the amount of dsDNA quantified by picoGreen (Life Technology). Oxygen consumption assay Oxygen consumption was measured in CeMM with lab-made respirometers ( Fig. 5b ) [43] . Synchronized L1 larvae were carefully titrated and ~15,000 worms were transferred to a CeMM agar chunk. The chunk was placed in the lid of the respirometer. The respirometer contains soda lime, which absorbs expelled CO 2 and thus decreases the pressure. The change in gas volume (decreased pressure) is measured by the displacement of fluid in a glass capillary attached to the closed respirometer. Nile red staining Newly hatched L1 larvae were grown on CeMM or OP50 for 2 h, then fixed in 40% isopropanol at room temperature for 3 min and stained in Nile Red working solution in dark for 2 h. Worms were then washed with PBS (0.01% Triton-X-100 included) for at least 30 min, mounted on slides and imaged under the green fluorescent protein channel of microscope. Fluorescent density was measured using Image J software. More than 10 animals from each experiment ( n ) were used to calculate the fluorescent density. Behavioural assays For male mating potency in NGM E. coli OP50 plates, each 1-day-old male was put onto an individual plate with a 5–10 mm lawn of OP50 containing a 1-day-old fog-2(q71) female. Successful mating was scored if there was at least 1 progeny 24 h later. For male mating potency on CeMM, each 1-day-old male was put onto an individual CeMM 1.7% agarose well in a 24-well tissue culture plate, with six 1-day-old fog-2(q71) female. The virgin 1-day-old males were either grown in OP50 plates or in CeMM plates. Successful mating was scored if there were progeny 24 h days later. For spicule insertion efficiency assays on CeMM, 10 2-day-old unc-64(e246) adult hermaphrodites were put onto a 5-mm-diameter area of a CeMM plate. Each 1-day-old male was placed in the centre of the hermaphrodite group, using a glass capillary pipette and water as a vehicle. These 1-day-old males either were grown on CeMM plates or on OP50 plates, separated from hermaphrodite siblings at L4 stage to new respective plates for about 20 h. As adults, they were transferred to a CeMM plate, where they were allowed to acclimate for an hour before the assay. We placed the mating groups on an Olympus SZX16 stereomicroscope mounted with a Hamamatsu ImagEM CCD camera. The efficiency of spicule insertion, ESI, was calculated from recordings made during the first 120 s of contact between the male and a paralyzed 2-day-old hermaphrodite. The metrics recorded were: (1) duration of prodding at the vulva; (2) duration in contact with other areas of the hermaphrodite. Recordings were stopped if the male inserted his spicules within the 120-s assay period. ESI=(time (s) spent at spicule insertion attempts/total time (s) in contact with hermaphrodite, up to 120 sec) × (1/time (s) in contact with the hermaphrodite, such as scanning, but not attempting insertion (penalty)) × (1+(0 if no penetration, otherwise time (s) remaining after a successful penetration, /120 s)(bonus)). To assay mating drive, according to ‘Tendency to Copulate Assay’ from Emmons’ group with modification, 10 2-day-old immobile unc-64(e246) adult hermaphrodites were put onto a 5-mm-diameter bacterial lawn. Each 1-day-old male was placed outside of the bacterial lawn with a mouth pipette and water as a vehicle. In a 10-min observation period, the duration required for the male to contact and start mating with the hermaphrodite, after he enters the bacterial lawn, was measured. How to cite this article: Zhang, L. et al . TMC-1 attenuates C. elegans development and sexual behaviour in a chemically defined food environment. Nat. Commun. 6:6345 doi: 10.1038/ncomms7345 (2015).